Beating beats mixing in heterodyne detection schemes Heterodyne detection schemes are widely used to detect and analyse high-frequency signals, which are unmeasurable with conventional techniques. It is the general conception that the heterodyne signal is generated only by mixing and that beating can be fully neglected, as it is a linear effect that, therefore, cannot produce a heterodyne signal. Deriving a general analytical theory, we show, in contrast, that both beating and mixing are crucial to explain the heterodyne signal generation. Beating even dominates the heterodyne signal, if the nonlinearity of the mixing element (mixer) is of higher order than quadratic. The specific characteristic of the mixer determines its sensitivity for beating. We confirm our results with both a full numerical simulation and an experiment using heterodyne force microscopy, which represents a model system with a highly non-quadratic mixer. As quadratic mixers are the exception, many results of previously reported heterodyne measurements may need to be reconsidered. There are many periodic processes with such a high frequency that they are difficult to measure experimentally. A solution is the application of a heterodyne detection scheme, as it down-converts the high-frequency signal to a lower, easily measurable frequency by mixing it with a reference signal. This enables the quantification of the amplitude, the phase and the frequency modulation of the original, high-frequency signal. A well-known example of a heterodyne detector is the radio. Heterodyne detection is also widely used in optics, in quantum devices, in the detection of nuclear magnetic resonance, in microwave detection, in scanning tunnelling spectroscopy and even in the search for gravitational waves [1] , [2] , [3] , [4] , [5] , [6] , [7] . Despite the successful application of heterodyne detection schemes, the exact generation of the heterodyne signal is often not well understood such that quantitative interpretations are only possible with extensive numerical calculations. Moreover, until now it has not been realized that the standard textbook equation for mixing usually fails, as in reality almost all mixers contain a beating stage at their input. To address this problem, we derived a general analytical theory that uses beating plus mixing for the generation of the heterodyne signal such that it becomes valid for all heterodyne detection schemes. Although not recognized, almost all heterodyne mixers have a single input channel, through which a superposition is realized of the high-frequency signal and the reference signal before the real nonlinear mixing takes place: in optics, for example, the measured intensity is the square of the superposed electric fields. Consequently, we have to differentiate between beating, which is a linear effect occurring for superpositions and mixing occurring for nonlinear couplings. In the following, we show that both beating and mixing are necessary to correctly describe the generation of the heterodyne signal. By deriving a general analytic theory that we confirm with simulations and experiments, we demonstrate that beating plays a crucial role in any type of heterodyne measurement system. In particular, we show that beating dominates mixing, if the mixer is of higher order than quadratic. Differentiating between Beating and Mixing The upper panel of Fig. 1 depicts beating: it is the sum of two harmonic excitations at frequencies ω s and ω t . The result (black line) oscillates with a frequency ω h ( ω s < ω h < ω t ) and beats in amplitude at the difference frequency ω diff = |ω s − ω t | (red lines). However, as the Fourier transform of the time trace only shows the two original frequencies ω s and ω t , no signal is generated at the difference frequency ω diff . Mixing, see lower panel of Fig. 1 , is the product of two or more harmonic excitations and occurs if the transfer function of the mixer is of quadratic or higher order. This result really oscillates at the difference frequency (red line) and the sum frequency (black line). In contrast to beating, the Fourier transform shows the difference and the sum frequency, but not the two frequencies of the original harmonic excitations. Although beating and mixing are two intrinsically different effects that are classified by the type of mixer and their Fourier analyses, we will fully counterintuitively demonstrate that beating even dominates mixing, if the mixer is of higher order than quadratic! 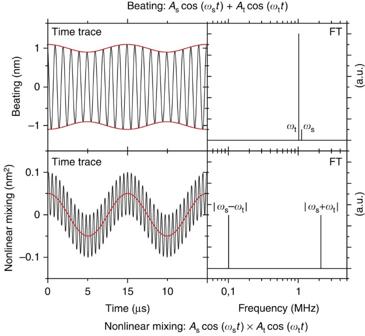Figure 1: Beating versus mixing. Beating is the sum of two harmonic functions (upper panel): the Fourier transform (FT) contains only the two original frequenciesωsandωt. Mixing is the product of two harmonic functions (lower panel): the FT contains only the two nonlinear frequencies|ωs−ωt| and |ωs+ωt|. The graphs have been calculated forωs=1.1 MHz,ωt=1 MHz,As=0.1 nm andAt=1 nm. Figure 1: Beating versus mixing. Beating is the sum of two harmonic functions (upper panel): the Fourier transform (FT) contains only the two original frequencies ω s and ω t . Mixing is the product of two harmonic functions (lower panel): the FT contains only the two nonlinear frequencies |ω s − ω t | and | ω s + ω t |. The graphs have been calculated for ω s =1.1 MHz, ω t =1 MHz, A s =0.1 nm and A t =1 nm. Full size image To illustrate the importance of beating in heterodyne measurements, we use the example of heterodyne force microscopy (HFM) [8] , [9] , [10] , as it represents a model system with a highly nonlinear mixing element (much higher order than quadratic). HFM enables the non-destructive imaging below a surface with nanometre resolution using an atomic force microscope [11] , [12] , [13] , [14] , [15] , [16] , [17] , [18] , [19] . The typical excitation scheme is sketched in Fig. 2a . The subsurface information is contained in an ultrasonic sound wave that travelled through the sample with a frequency ω s of several MHz (well above the first resonance of the cantilever). To detect this signal, one applies a heterodyne detection scheme and excites, therefore, also the cantilever/tip with a high frequency ω t that deviates slightly from ω s . The nonlinear tip–sample interaction generates a heterodyne signal at a sufficiently low difference frequency ω diff such that the cantilever really starts to move at ω diff . In this way, the tip–sample distance is the superposition of the sample vibration with amplitude A s and phase φ s , and the cantilever vibration with amplitude A t and phase ϕ t , on the basis of which the nonlinear tip–sample interaction generates the difference frequency. Usually, one tunes ω diff below the first resonance of the cantilever, however, this choice is not necessary, as long as the difference frequency can still excite a real motion in the cantilever. This information is provided by the transfer function of the cantilever, as it describes the reaction of the cantilever for a given applied force as a function of the frequency. 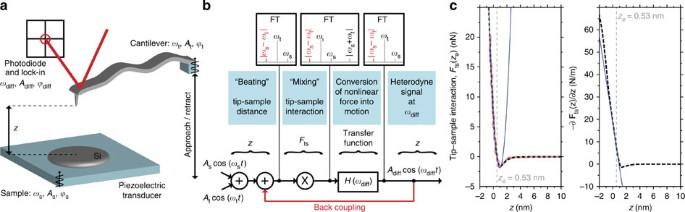Figure 2: Heterodyne force microscopy excitation scheme. (a) The Si sample vibrates with amplitudeAsand phaseϕsat a frequencyωs, while the tip vibrates withAtandϕtatωt. Using an optical beam method and a lock-in, we detected the amplitudeAdiffand phaseϕdiffof the difference frequencyωdiff=|ωs−ωt|. The tip–sample distancezwas varied by moving the cantilever towards the surface (approach) and out again (retract). (b) The tip–sample distance is the sum of the ultrasonic motion of the cantileverAtcos(ωtt) and the sampleAscos(ωst), which results in beating. The nonlinear tip–sample interaction generates drive forces (among others at the difference frequency), which lead, via the transfer functionH(ωdiff) of the cantilever that also acts as a low-pass filter, to a real motion that is coupled back into the tip–sample distance (red arrow). (c) The tip–sample interaction as a function of the distancez(left panel): obtained from the experiment (red), as used in the analytical calculation (dashed black), and a second-order approximation aroundze=0.53 (blue). The derivative of the tip–sample interaction as a function of the distancez(right panel): as used in the analytical calculation (dashed black) and the second-order approximation aroundze=0.53 (blue). The blue line is only a good approximation ofFtsnearz=ze=0.53. Figure 2: Heterodyne force microscopy excitation scheme. ( a ) The Si sample vibrates with amplitude A s and phase ϕ s at a frequency ω s , while the tip vibrates with A t and ϕ t at ω t . Using an optical beam method and a lock-in, we detected the amplitude A diff and phase ϕ diff of the difference frequency ω diff = |ω s −ω t |. The tip–sample distance z was varied by moving the cantilever towards the surface (approach) and out again (retract). ( b ) The tip–sample distance is the sum of the ultrasonic motion of the cantilever A t cos( ω t t ) and the sample A s cos( ω s t ), which results in beating. The nonlinear tip–sample interaction generates drive forces (among others at the difference frequency), which lead, via the transfer function H ( ω diff ) of the cantilever that also acts as a low-pass filter, to a real motion that is coupled back into the tip–sample distance (red arrow). ( c ) The tip–sample interaction as a function of the distance z (left panel): obtained from the experiment (red), as used in the analytical calculation (dashed black), and a second-order approximation around z e =0.53 (blue). The derivative of the tip–sample interaction as a function of the distance z (right panel): as used in the analytical calculation (dashed black) and the second-order approximation around z e =0.53 (blue). The blue line is only a good approximation of F ts near z = z e =0.53. Full size image Figure 2b depicts the heterodyne signal generation for the example of HFM. The sum of the ultrasound signals at frequencies ω t and ω s results in beating at the mixer’s input. This mixer generates a heterodyne drive force at ω diff , which results in a real motion of the cantilever via the cantilever’s transfer function H ( ω diff ). HFM is special, as the output of this transfer function (real motion at ω diff ) is coupled back into the tip–sample distance, which leads to an additional beating term at the input of the mixer. The transfer function also acts as a filter, which eliminates almost any contribution from the sum frequency | ω t + ω s |, as well as higher-order mixing terms: A | ω s + ω t | / A | ω s + ω t | =0.004 . We derive the transfer function in Supplementary Note 5 . We also address the general case without back coupling to the mixer below, as well as in Supplementary Note 4 , and show that beating still gives significant corrections to the heterodyne signal. Although the back coupling can, in principle, also alter the ultrasonic amplitudes A t and A s (and corresponding phases), it was surprisingly shown experimentally that A t and A s remain constant for all tip–sample distances z in HFM [20] , [21] . Therefore, HFM behaves exactly as a conventional heterodyne detection scheme with an additional back coupling of only the difference frequency signal ω diff =| ω s − ω t | to the input of the mixer. Analytical theory for the heterodyne signal generation To derive an expression for the heterodyne signal, we need a description of the mixer’s input, which is given by the tip–sample distance z . This distance contains a static offset z b given by the position of the cantilever’s base, a deflection δ and a back coupling term that accounts for the real motion at the difference frequency, in addition to the ultrasonic motion of both the cantilever and the sample. To enable a proper comparison between our theory and both a numeric simulation and experiments, we subtract an offset in z b such that z b =0, if the deflection δ =0 during the approach cycle of the cantilever to the surface. Equation (1) is used for the input signal of the mixer, which generates via the nonlinear tip–sample interaction F ts ( z ) an effective drive force on the cantilever at the difference frequency. The derivation can be performed in two ways: either one makes, as usual, a second-order Taylor expansion of the tip–sample interaction around the equilibrium position (which is z e = z b + δ ) or one first uses beating to rewrite the high-frequency components of the mixer’s input as a motion at a high frequency ω h with amplitude and an additional amplitude modulated term at the same frequency, before making a linear expansion of the tip–sample interaction around a time varying equilibrium position. This linear expansion is justified, as a third-order expansion alters the heterodyne signal at most by 4.5%. The first method, referred to as ‘Standard Mixing’ can be found in most textbooks, but (commonly not mentioned) this solution is valid only for second-order (quadratic) interactions. In contrast, our alternative approach, which we call ‘Beating & Mixing’, is valid for any type of interaction. The derivations and validities of both methods are described in detail in Supplementary Notes 2–4 . ‘Beating & Mixing’ is a generalization of the standard theory and produces the ‘Standard Mixing’ results, if one artificially sets the beating term to zero. We find proof for our ‘Beating & Mixing’ description from excellent agreements of our results from numerical simulations and HFM experiments, as discussed below. Let us now compare the ‘Standard Mixing’ textbook solution with our ‘Beating & Mixing’ generalization, in which the amplitude A diff and the phase ϕ diff of the heterodyne signal ( Table 1 ; equation (2)) and the static deflection δ of the cantilever ( Table 1 ; equation (3)) are determined by three parameters: I 0 denotes the average tip–sample interaction, I 1 denotes an effective tip–sample spring and I 2 represents the nonlinear characteristics (curvature) of the mixer. In the ‘Standard Mixing’ solution, I 1 and I 2 are determined by the values of the first and the second derivative of the tip–sample interaction at the equilibrium position z e . In contrast, the ‘Beating & Mixing’ solution takes explicitly into account the high-frequency motion and, therefore, the derivative of the tip–sample interaction at all tip–sample distances between z e and z e ± A h . This description holds as long as A s · A t is smaller than A h 2 . The three parameters I 0 , I 1 and I 2 become weighted integrals of F ts and ∂F ts /∂z . Only if the mixer is purely quadratic, the integrals reduce to the exact values for I 0 , I 1 and I 2 of the textbook solution of ‘Standard Mixing’ (see Supplementary Note 3 ). Consequently, the ‘Beating & Mixing’ solution is required for all mixers that cannot be approximated with a quadratic function. Table 1 Analytical expressions for the heterodyne signal. Full size table The tip–sample interaction in HFM deviates significantly from a quadratic behaviour. This becomes evident from the left panel of Fig. 2c , in which we show F ts obtained from the experiment (red), F ts as used in the analytical calculation (dashed black) and the quadratic interaction or second-order approximation of F ts around z = z e =0.53 nm (blue). Although the quadratic interaction is a good approximation of the tip–sample interaction close to z e =0.53 nm, this approximation clearly fails 1 nm further at a tip–sample distance of, for example, z = z e =1.53 nm. This is even worse for the first derivative of the tip–sample interaction, which is shown in the right panel of Fig. 2c . Therefore, ‘Standard Mixing’ cannot describe the heterodyne signal generation in HFM: the tip–sample interaction cannot be approximated quadratically over a z range that is equal to the typical ultrasonic vibration amplitude A h of 1 nm. Experimental verification of the ‘Beating & Mixing’ theory In Fig. 3 , we compare the ‘Beating & Mixing’ result with a full numerical simulation, an experiment, and the ‘Standard Mixing’ theory. For simplicity, we only show the approach curves. Both the ‘Beating & Mixing’ theory and the ‘Standard Mixing’ theory, as well as the numerical simulation, need an analytical description of the tip–sample interaction, which we obtained by fitting the Derjaguin–Muller–Toporov model [22] and I 0 to the experimental deflection δ (see Supplementary Note 6 ). This experiment was performed with a 2 N m −1 cantilever, which had its first resonance frequency around 73 kHz. The sample was a freshly cleaned silicon wafer. The cantilever was excited at 2.87 MHz with an amplitude of 0.96 nm, while the sample was excited such that ω diff =1 kHz. The vibration amplitude of the sample was 0.32 nm. The full experimental details are described in Supplementary Note 7 . 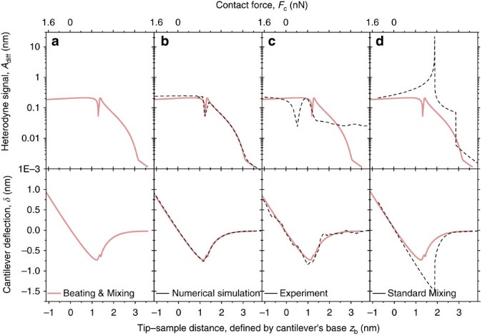Figure 3: Comparison between analytical theory, simulation, and an experiment. The heterodyne amplitudeAdiffas obtained from ‘Beating & Mixing’ (a: red), from a full numerical simulation (b: black), from the experiment (c: black) and from ‘Standard Mixing’ (d: black). For comparison, the ‘Beating & Mixing’ curves (red) are also shown inb,candd. The bottom panels show the corresponding static deflectionδof the cantilever. Notice that both the numerical simulation and the experimental results support the validity of ‘Beating & Mixing’: their curves qualitatively fit the ‘Beating & Mixing’ ones. In contrast, ‘Standard Mixing’ deviates significantly. Figure 3: Comparison between analytical theory, simulation, and an experiment. The heterodyne amplitude A diff as obtained from ‘Beating & Mixing’ ( a : red), from a full numerical simulation ( b : black), from the experiment ( c : black) and from ‘Standard Mixing’ ( d : black). For comparison, the ‘Beating & Mixing’ curves (red) are also shown in b , c and d . The bottom panels show the corresponding static deflection δ of the cantilever. Notice that both the numerical simulation and the experimental results support the validity of ‘Beating & Mixing’: their curves qualitatively fit the ‘Beating & Mixing’ ones. In contrast, ‘Standard Mixing’ deviates significantly. Full size image To confirm that ‘Beating & Mixing’ is important in HFM, we calculated both the amplitude of the heterodyne signal A diff and the deflection δ as a function of the tip–sample distance (defined by the cantilever’s base position z b ; see Fig. 3a ). The numerical simulations quantitatively fit our ‘Beating & Mixing’ curves (see black line in Fig. 3b ) perfectly. Additional proof comes also from experiments (see Fig. 3c ) [21] , as the general curvature correctly reproduces the ‘Beating & Mixing’ results at all tip–sample distances z b . If we compare the textbook solution of ‘Standard Mixing’ shown in Fig. 3d , one clearly notices a significant deviation: ‘Standard Mixing’ fails to describe the mixing signal. This is in contradiction with the general conception that standard frequency mixing generates the observed signal in HFM. The discontinuities, in both the amplitude and the deflection, are due to the specific choice of tip–sample interaction (see Supplementary Note 6 ). In conclusion, this confirms that ‘Beating & Mixing’ indeed correctly describes the generation the difference signal in HFM and that ‘Standard Mixing’ fails. Let us now discuss the significant effect of the ultrasound on the deflection in HFM, which can be evaluated by the static output ( I 0 ) of the mixer with respect to the case without ultrasound. Alternatively, one can compare the deflection curves of the ‘Standard Mixing’ theory with the ‘Beating & Mixing’ theory, which is shown in Fig. 3d . In conclusion, both the adhesion and the elasticity appear smaller in HFM experiments, if one does not account for the existence of the ultrasound. Finally, we address the more general case of heterodyne measurements without a back coupling to the input of the mixer as existent in HFM. Even without back coupling, beating is still essential to correctly describe the heterodyne signal generation. As the back coupling term in HFM is generated by I 1 (see Supplementary Note 4 ), we can set I 1 to zero in equation (2). Also without back coupling, ‘Beating & Mixing’ still determines the heterodyne signal and the static deflection through the parameters I 0 and I 2 . Therefore, we generally conclude that beating is of crucial importance for heterodyne detection schemes. In conclusion, we have shown that beating, although it is a linear effect and has never considered to be of importance in heterodyne detection schemes, dominates the generation of the signal at the difference frequency in heterodyne measurements. We derived a general, analytical theory for any type of interaction that takes into account Beating & Mixing, and shown that our ‘Beating & Mixing’ theory correctly produces the standard beating solution for a pure linear interaction, as well as the Standard Mixing solution for an interaction that is purely quadratic. Correction terms are necessary for any interaction that is of higher order than quadratic. We verified our theory with a finite time step simulation and with an experiment applying HFM, which is a typical example of a heterodyne measurement with a highly non-quadratic mixer. How to cite this article: Verbiest, G. J. and Rost, M. J. Beating beats mixing in heterodyne detection schemes. Nat. Commun . 6:6444 doi: 10.1038/ncomms7444 (2015).